Model-based identification of drug targets that revert disrupted metabolism and its application to ageing The growing availability of ‘omics’ data and high-quality in silico genome-scale metabolic models (GSMMs) provide a golden opportunity for the systematic identification of new metabolic drug targets. Extant GSMM-based methods aim at identifying drug targets that would kill the target cell, focusing on antibiotics or cancer treatments. However, normal human metabolism is altered in many diseases and the therapeutic goal is fundamentally different—to retrieve the healthy state. Here we present a generic metabolic transformation algorithm (MTA) addressing this issue. First, the prediction accuracy of MTA is comprehensively validated using data sets of known perturbations. Second, two predicted yeast lifespan-extending genes, GRE3 and ADH2 , are experimentally validated, together with their associated hormetic effect. Third, we show that MTA predicts new drug targets for human ageing that are enriched with orthologs of known lifespan-extending genes and with genes downregulated following caloric restriction mimetic treatments. MTA offers a promising new approach for the identification of drug targets in metabolically related disorders. The traditional paradigm for drug discovery faces growing difficulties in meeting the need for new medicines that can cure, prevent or slow the progression of disease. Evidently, the discovery of new and better drug targets is a key in transforming industry productivity and in bringing innovative new medicines to patients. In particular, systems biology is suggested as a promising approach for aiding the drug discovery process [1] . The growing availability of genome-wide high-throughput molecular screens, together with high-quality in silico models of cellular metabolism, provides a golden opportunity for the rational and systematic identification of new metabolic drug targets. Here we present a novel metabolic transformation algorithm (MTA) for identifying drug targets in genome-scale metabolic networks. As opposed to existing methods that search for drug targets that would kill the target cell [2] , [3] , MTA aims to identify targets that would act to alter the metabolism of the cell, in a manner that would retrieve it back from a given disease state to a healthier state. MTA utilizes a GSMM and gene expression measurements of a given source (disease) and a target (healthy) metabolic state. To guide its prediction, MTA analyses the differences in gene expression between the two states and determines the desirable global change in the network. On the basis of that signature, MTA then searches for the genetic or environmental perturbations that best enable a transformation from the source to the target state. The MTA algorithm is based on GSMM, an increasingly widely used computational framework for studying metabolism on a genome-scale. Given a species’ GSMM and pertaining contextual information such as the growth media and ‘omics’ data, one can harness a constraint-based modeling (CBM) approach to impose a set of context-specific constraints on the space of possible metabolic behaviours, and obtain a fairly accurate prediction of numerous metabolic phenotypes, including growth rates, nutrient uptake rates, by-product secretion and gene essentiality (see ref. 4 ). GSMMs have been used for a variety of applications [5] , [6] , [7] , [8] , [9] , [10] including drug discovery [2] and metabolic engineering tasks [11] . Over the last 6 years, GSMM has been successfully used for modelling human metabolism as well, both in health and disease [3] , [12] , [13] , [14] , [15] , [16] . The numerous arising applications of GSMMs for identifying drug targets, both in pathogens and in human disease, have been recently comprehensively reviewed in refs 2 , 17 , 18 . Several GSMM methods for predicting the phenotypic effects of gene perturbations have been developed and successfully used in microorganisms. To predict these effects, the said approaches rely on a predefined cellular objective function, such as the maximization of growth rate or the minimal amount of flux changes with respect to the source metabolic state [19] , [20] . Here we address a related, yet a more challenging goal: as MTA’s aim is to find perturbations that would alter the metabolism of diseased cells, many of which are non-proliferating, its predictions cannot be guided by a predefined objective function of such cells that is both unknown for most non-proliferating tissues/cells, and may vary from one tissue to another. Instead, MTA exploits the measured gene expression of the desired target state and aims to identify the perturbations that will most probably bring the network from a given source state to a state that is as close as possible to this desired target state. By considering this additional information on the target state MTA goes beyond current drug target prediction GSMM methods, suggesting a fresh new approach for identifying novel metabolic drug targets. A classical biological process in which perturbations are known to at least partially transform a source state into a target one is ageing. ageing is typically accompanied by genome-wide changes in gene expression where lowered expression of metabolic and biosynthetic genes has a key role [21] . Interestingly, it has been shown that caloric restriction (CR), a dietary intervention that reliably extends lifespan, opposes the development of many of these age-associated gene expression changes [22] . Although CR is of limited utility therapeutically, these findings have strongly motivated the search for agents that work analogously to CR by counteracting metabolic alterations in ageing. These interventions include the insulin-like growth factor 1 (ref. 23 ), the sirtuin proteins [24] , [25] , resveratrol [26] and the mammalian target of rapamycin [27] . Accordingly, ageing data sets serve as a promising test bed for MTA in identifying perturbations, both genetic and environmental, that can potentially transform an aged metabolic state towards the desired younger one, and thus work to extend the organism’s lifespan. In the following, we first introduce MTA and validate its predictive ability across numerous published perturbation experiments in different species, where the underlying perturbation is known but hidden from the algorithm. Second, we apply MTA to predict lifespan-extending genes in yeast, a key model of cellular ageing, experimentally validating two predicted metabolic genes whose knockout leads to a marked increase in yeast lifespan. Following a model-based hypothesis, we further show experimentally that the knockout of these two predicted target genes results with higher levels of reactive oxygen species (ROS) production, suggesting a hormetic effect that leads to lifespan extension. Finally, MTA is applied to predict metabolic drug targets that most efficiently transform the metabolic state of ageing human muscle tissue back closer to its young state, and its predictions are reassuringly enriched with known human orthologs of known lifespan-extending genes. Although it has been developed and studied here in the context of ageing, it is evident that MTA has a much wider scope of potential applications, aimed at identifying perturbations that can revert the disease state back closer to a healthy one in a variety of metabolically related disorders. The MTA Our goal is to develop a computational approach that will enable a systematic search for all reactions/genes whose perturbation can induce a transformation of the metabolic state from a given source state (for example, diseased) to a desired target state (for example, a healthy one), as much as possible. The MTA, a generic approach designed to this end, receives as input a GSMM of a certain species, together with gene expression levels measured under source and target states. The algorithm then proceeds in four steps: (1) a flux description of the source metabolic state is obtained by utilizing a published CBM method termed integrative metabolic analysis tool (iMAT) [14] , which integrates the gene expression levels measured in the source state to predict a most likely distribution of metabolic fluxes (see Methods ). (2) two sets of reactions are identified: (a) those significantly differing in their gene expression levels between the source and target states (termed changed reactions) and (b) those reactions whose gene expression levels are not significantly altered between states (termed unchanged reactions). Ideally, MTA seeks a perturbation that will successfully shift all the fluxes of the changed reactions in the right direction while keeping the fluxes of the unchanged reactions as close as possible to the source state. (3) Next, to find the best ‘transforming’ knockout reactions, all the reactions in the network are individually perturbed at the source state one at a time (for instance, by forcing their flux to zero), and the potential of the network to obtain the desired shift to the target state under each perturbation is examined. This step is performed using a new mixed integer quadratic programming (MIQP) algorithm that maximizes the number of changes in the changed class while minimizing the changes in the unchanged class (identified in step (2)). (4) A transformation score (TS) is assigned to each perturbation simulated in step (3), reflecting the extent by which it may transform the source state to the target flux state. The perturbations are then ranked according to their scores (see Fig. 1 for an overview of the computational approach). 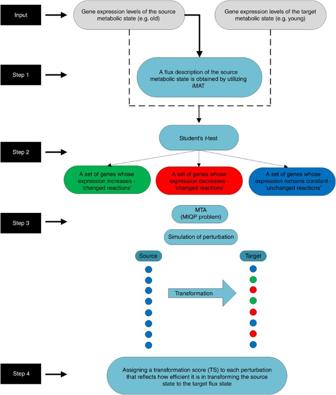Figure 1: A schematic overview of MTA. MTA aims to find perturbations that are most likely to result with a successful transformation from a given source metabolic state to a desired target state. MTA is described above at the reactions’ level, where a perturbation refers to shutting down the flux in the pertaining reaction, but can also be performed on the gene level using the gene-protein-reaction mapping embedded in each GSMM. Figure 1: A schematic overview of MTA. MTA aims to find perturbations that are most likely to result with a successful transformation from a given source metabolic state to a desired target state. MTA is described above at the reactions’ level, where a perturbation refers to shutting down the flux in the pertaining reaction, but can also be performed on the gene level using the gene-protein-reaction mapping embedded in each GSMM. Full size image Validating MTA through data sets of known perturbations To examine the performance of MTA, we first applied it to predict the effects of gene knockouts in Escherichia coli , mouse and human data sets ( Supplementary Tables S1 and S3 ). These data sets contain gene expression data measured before and after a specific metabolic gene knockout, providing a test bed for MTA. That is, given the organism’s metabolic model and the pertaining wild-type and knockout gene expression measurements, MTA’s goal is to correctly identify the gene knockout steering this specific metabolic transformation from the wild-type into the knockout state, which is known but ‘hidden’ from the algorithm. Of note, although the prime task of MTA is to identify perturbations transforming a diseased state back to a healthy one, it is formulated in a completely generic manner that enables one to identify transforming perturbations between any given source and target states. As depicted in Fig. 2a , the true underlying knockouts are ranked very highly, and within the top 10% of MTA’s predictions (Bernoulli’s test, P -value=1e−15, Supplementary Tables S1,S3 and S4 ). To further test MTA’s utility for other types of perturbations, we applied it to predict environmental perturbations in E. coli and yeast as well ( Supplementary Tables S1,S2 ). Namely, given a pair of gene expression samples measured under two different carbon sources, we examined its ability to correctly predict the specific carbon source used in the new growth media (Methods). As depicted in Fig. 2b, this analysis yields a high predictive performance as well (Bernoulli’s test, P -value<2.2e−16, Supplementary Tables S1,S2 and S4 ). To further study the nature of our algorithm, we examined the alternative top-ranked reactions suggested by MTA in various experiments. Indeed, in many cases when the underlying reaction is not ranked at the top of the list, this is because there are several other reactions whose knockout has identical functional effects in the model and are hence as likely to be identified as the specific reaction perturbed (see Supplementary Fig. S1 ). For comparison, applying existing knockout prediction CBM algorithm such as the widely used minimization of metabolic adjustment (MOMA) method [20] results with markedly inferior performance (Methods and Supplementary Tables S1–S3 ). Further, it should be emphasized that in most of the experiments used here, the underlying perturbation could not have been gleaned from the gene expression signatures themselves ( Supplementary Table S5 ). 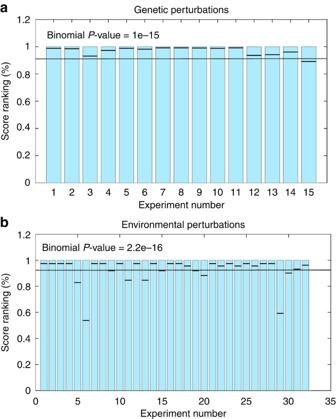Figure 2: Bar plots summarizing MTA’s perturbation validation analysis. (a) The left panel describes the results obtained for gene knockouts data sets, where bars 1–11 correspond to data measured inE. coli, bars 12–13 correspond to mouse and 14–15 correspond to human cells. The horizontal bars represent the computed ranking of the actual knockout that has been performed in the experiment (normalized here to a value in the range [0 1]) amongst all other simulated knockouts. In all cases, the correct knockout is ranked within the top 10% predictions (dashed line, Bernoulli’s test,P-value=1e−15 withP=0.1). (b) The right panel presents the results obtained under environmental perturbations (the switching of carbon sources in the growth media, simulated by inhibiting the corresponding transport reactions), where bars 1–29 describe the results forE. coliand bars 30–32 for yeast. In 26 of the 32 experiments examined, the correct carbon source that has been used in the experiment is ranked within the top 10% predictions (Bernoulli’s test,P-value<2.2e−16 withP=0.1). A detailed listing of the experiments analysed and of the predictions made by MTA is provided inSupplementary Tables S1–S3. Figure 2: Bar plots summarizing MTA’s perturbation validation analysis. ( a ) The left panel describes the results obtained for gene knockouts data sets, where bars 1–11 correspond to data measured in E. coli , bars 12–13 correspond to mouse and 14–15 correspond to human cells. The horizontal bars represent the computed ranking of the actual knockout that has been performed in the experiment (normalized here to a value in the range [0 1]) amongst all other simulated knockouts. In all cases, the correct knockout is ranked within the top 10% predictions (dashed line, Bernoulli’s test, P -value=1e−15 with P =0.1). ( b ) The right panel presents the results obtained under environmental perturbations (the switching of carbon sources in the growth media, simulated by inhibiting the corresponding transport reactions), where bars 1–29 describe the results for E. coli and bars 30–32 for yeast. In 26 of the 32 experiments examined, the correct carbon source that has been used in the experiment is ranked within the top 10% predictions (Bernoulli’s test, P -value<2.2e−16 with P =0.1). A detailed listing of the experiments analysed and of the predictions made by MTA is provided in Supplementary Tables S1–S3 . Full size image Predicting lifespan-extending metabolic targets in yeast The budding yeast Saccharomyces cerevisiae is a widely used model of cellular ageing. Although it is a single-celled eukaryote, increasing evidence show that longevity pathways in yeast are conserved in other multicellular eukaryotes [28] . To further test the predictive power of MTA, we applied it to analyse gene expression data of young and ageing yeast from an assay examining their replicative lifespan (RLS) [29] , and from an assay examining their chronological lifespan (CLS) [30] . For each of these data sets separately, we predicted a set of reactions whose individual knockout can transform the aged metabolic state towards that of the young. Remarkably, this set was found to be significantly enriched with genes whose knockout is known to extend the yeast’s lifespan (termed lifespan-extending genes), collected from the Sacchromyces Genome Database (SGD) and from the literature [28] , [31] , [32] , [33] (Permutation test, empirical P -value<0.03, both for RLS and CLS, see Supplementary Data 1 ). After reviewing the list of MTA’s top predictions (for example, HXK2/YGL253W, TGL3/YMR313C and FCY2/YER056C , see Supplementary Data 1 ) and excluding genes that were shown to be involved in CLS based on the list compiled above, we chose seven novel gene targets for further experimentation. Genes were chosen based on their high ranking in the prediction list, representing distinct metabolic pathways, and existing in a single isoform ( Supplementary Table S6 ). For yeast CLS measurements, the cells were grown to stationary phase in liquid media and the percentage of viable cells was measured periodically by determining the fraction of viable cells capable of forming a colony when plated onto rich media. Out of these, two gene knockouts, gre3Δ and adh2Δ, were found to significantly extend yeast’s median lifespan, with gre3Δ extending median lifespan by ~100% (Wilcoxon’s test, P -value=8.22e–5 and 1.65e–4 for gre3Δ and adh2Δ, respectively, Fig. 3a , Methods and Supplementary Fig. S2 ). Although GRE3 was previously found to be downregulated in a sir2Δ strain, it is further validated here as having a causative role as lifespan-extending gene [34] . Overall, this result constitutes a 10-fold increase over the expected frequency, as only 3.5% of the yeast genes are expected to extend CLS by random (Bernoulli’s test, P -value=0.02, Methods) [33] . Of note, the ranking obtained by MOMA or the gene expression alone to the above genes is again markedly inferior ( Supplementary Table S6 ). 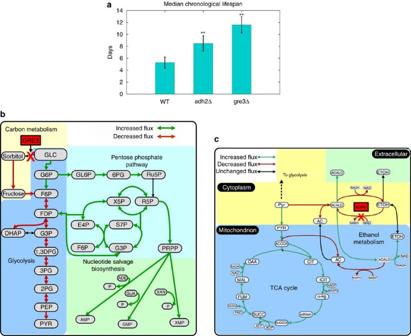Figure 3: Extension of yeast CLS by predicted genes. (a) Median CLS (in days) for the wild-type (WT), adh2Δ and gre3Δ strains. A significant increase in the median lifespan is observed for gre3Δ and adh2Δ strains (Wilcoxon’s test,P-value=8.22e−5 andP-value=1.65e−4, respectively). Error bars represent the s.d. (n=3). Each of the platings was done in triplicate and three distinct colonies of each strain were tested. (b) Guided by changes in gene expression associated with a decrease in the nucleotide salvage pathway and purine and pyrimidine biosynthesis, MTA correctly identifiesGRE3as a lifespan-extending gene. A stoichiometric analysis shows that this inhibition reduces the flux through glycolysis. The elevated glucose levels are diverted to the pentose phosphate pathway and consequently increase the flux through nucleotide synthesis. At the same time, a reduction in the maximal flux through the reactions that detoxify ROS via glutathione and thioredoxin is observed (not shown in the figure). (c) Following the knockout ofADH2, a reduction in the metabolic flux through fermentation and an increase in flux through the TCA cycle is observed, as reviewed in ref.66. Remarkably, the expression level ofGRE3andADH2is not significantly altered between the two states (old versus young), demonstrating the value of the MTA analysis. GLC, glucose; G6P, glucose-6-phosphate; F6P, fructose-6-phosphate; FDP, fructose-1,6-bisphosphate; G3P, glyceraldehyde-3-phosphate; DHAP, dihydroxyacetone-phosphate; 1,3-DPG, 1,3-bisphosphoglycerate; 3PG, 3-phosphoglycerate; 2PG, 2-phosphoglycerate; PEP, phosphoenolpyruvate; PYR, pyruvate; GL6P, 6-phosphogluconolactone; 6PG, 6-phosphogluconate; Ru5P, ribulose-5-phosphate; R5P, ribose-5-phosphate; X5P, xylulose-5-phophate; S7P, sedohptulose-7-phosphate; E4P, erythrose-4-phosphate; PRPP, 5-phospho-D-ribose-α-1-pyrophosphate; ACCOA, acetyl-CoA; CIT, citrate; ICIT, isocitrate; α–kg, α-ketoglutarate; sdhlam,S-succinyldihydrolipoamide; SUCCOA, succinyl-CoA; SUCC, succinate FUM, fumarate, MAL, malate; OAA, oxaloacetate; AC, acetate; ACALD, acetaldehyde; ETOH, ethanol; TCA, tricarboxylic acid. **P<1e-3 Figure 3: Extension of yeast CLS by predicted genes. ( a ) Median CLS (in days) for the wild-type (WT), adh2Δ and gre3Δ strains. A significant increase in the median lifespan is observed for gre3Δ and adh2Δ strains (Wilcoxon’s test, P -value=8.22e−5 and P -value=1.65e−4, respectively). Error bars represent the s.d. ( n =3). Each of the platings was done in triplicate and three distinct colonies of each strain were tested. ( b ) Guided by changes in gene expression associated with a decrease in the nucleotide salvage pathway and purine and pyrimidine biosynthesis, MTA correctly identifies GRE3 as a lifespan-extending gene. A stoichiometric analysis shows that this inhibition reduces the flux through glycolysis. The elevated glucose levels are diverted to the pentose phosphate pathway and consequently increase the flux through nucleotide synthesis. At the same time, a reduction in the maximal flux through the reactions that detoxify ROS via glutathione and thioredoxin is observed (not shown in the figure). ( c ) Following the knockout of ADH2 , a reduction in the metabolic flux through fermentation and an increase in flux through the TCA cycle is observed, as reviewed in ref. 66 . Remarkably, the expression level of GRE3 and ADH2 is not significantly altered between the two states (old versus young), demonstrating the value of the MTA analysis. GLC, glucose; G6P, glucose-6-phosphate; F6P, fructose-6-phosphate; FDP, fructose-1,6-bisphosphate; G3P, glyceraldehyde-3-phosphate; DHAP, dihydroxyacetone-phosphate; 1,3-DPG, 1,3-bisphosphoglycerate; 3PG, 3-phosphoglycerate; 2PG, 2-phosphoglycerate; PEP, phosphoenolpyruvate; PYR, pyruvate; GL6P, 6-phosphogluconolactone; 6PG, 6-phosphogluconate; Ru5P, ribulose-5-phosphate; R5P, ribose-5-phosphate; X5P, xylulose-5-phophate; S7P, sedohptulose-7-phosphate; E4P, erythrose-4-phosphate; PRPP, 5-phospho-D-ribose-α-1-pyrophosphate; ACCOA, acetyl-CoA; CIT, citrate; ICIT, isocitrate; α–kg, α-ketoglutarate; sdhlam, S -succinyldihydrolipoamide; SUCCOA, succinyl-CoA; SUCC, succinate FUM, fumarate, MAL, malate; OAA, oxaloacetate; AC, acetate; ACALD, acetaldehyde; ETOH, ethanol; TCA, tricarboxylic acid. ** P <1e-3 Full size image An important added value of our computational framework is its ability to go beyond predicting the relevant target and search for a mechanism that best explains the observed phenotype. Analysing the rewiring of fluxes in the network following the knockout of GRE3 , we find a significant increase in flux rates through the pentose phosphate pathway. Although higher levels of NADP/NADPH are produced in this pathway, this increase was accompanied by a reduction in flux through the reactions that detoxify ROS by glutathione and thioredoxin ( Fig. 3b ). A similar analysis for adh2Δ showed an increase in the maximal flux through the tricarboxylic acid cycle ( Fig. 3c ). We hence hypothesized that an increase in ROS production may accompany lifespan extension in these strains. To validate this prediction, we measured the intracellular levels of two common ROS, hydrogen peroxide (H 2 O 2 ) and superoxide (O 2 − ), using flow cytometry and appropriate probes (see Methods ). Indeed, in comparison with wild-type yeast cells, a mild but significant increase in H 2 O 2 and O 2 − concentrations was observed during the course of chronological ageing in both adh2Δ and gre3Δ ( T -test, P -value<0.05, Fig. 4 ). Of note, this finding is in accordance with the hormesis theory of ageing, suggesting that exposure to mild stress results in a positive effect on lifespan [35] . However, here we demonstrate only an association between elevated ROS levels and lifespan extension, and the putative causative role that elevated ROS may have in these strains’ lifespan extension requires further study. 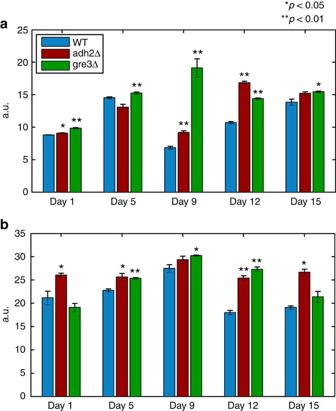Figure 4: Levels of ROS. Intracellular levels of two common ROS, H2O2(a) and O2−(b) measured during the course of the CLS assay. In comparison with WT yeast cells, a significant mild increase in both ROS levels was observed during the course of chronological ageing in both adh2Δ and gre3Δ strains (μ-test; *P<0.05; **P<0.01). Error bars represent the s.d.. Three replicates for ROS levels were examined in each strain. Figure 4: Levels of ROS. Intracellular levels of two common ROS, H 2 O 2 ( a ) and O 2 − ( b ) measured during the course of the CLS assay. In comparison with WT yeast cells, a significant mild increase in both ROS levels was observed during the course of chronological ageing in both adh2Δ and gre3Δ strains ( μ -test; * P <0.05; ** P <0.01). Error bars represent the s.d.. Three replicates for ROS levels were examined in each strain. Full size image Predicting metabolic targets counteracting muscle ageing To validate MTA in the context of human metabolism as well, we applied it to analyse gene expression data taken from four different data sets of human muscle tissue in old and young male and female subjects [36] , [37] , [38] , [39] ( Supplementary Fig. S3 ). As the sets of differentially expressed genes differ significantly between these data sets ( Supplementary Tables S7–S9 ), our validation is focused on the novel predictions of lifespan-extending gene knockouts in humans appearing in the top 10% of MTA’s predictions in at least two of the data sets (termed common knockout predictions, Supplementary Data 2 ). Top predicted reactions can reverse a significant portion of the ageing-related changes in all data sets (between 40 and 70% of the observed changes). Encouragingly, most of the predicted knockouts do not reduce the estimated maximal production of key currency metabolites that are generally conceived as essential to normal tissue functioning, such as ATP, NADP and NADPH (Methods and Supplementary Data 3 ). Of note, as CBM analysis does not allow the calculation of metabolites’ concentration, these values serve as only a rough approximation for the effect the predicted knockout may have on these metabolites’ production. Performing a cross-validation analysis amongst the individual samples composing each data set, the knockout predictions remain highly robust ( Supplementary Table S10 ). Reassuringly, the intersection between MTA’s predictions across the different data sets is mostly significant, thus suggesting a common metabolism-altering signature. Indeed, this intersection vanishes when the data are randomized ( Supplementary Tables S11,S12 ). As a first validation test, we examined whether our common knockout predictions set is enriched with genes whose expression is significantly reduced ( t -test, P -value<0.05) following CR mimetic treatments. To this end, we analysed gene expression data from muscle tissue of mice treated with resveratrol, rapamycin and those overexpressing the transcriptional co-activator PGC1- α (refs 26 , 40 ). As shown in Fig. 5a , a highly significant enrichment for all treatments was found (Hypergeometric test, P -value<9.99e–5). Further, we find that MTA’s common predictions set is enriched with human orthologs of known lifespan-extending genes in yeast and Caenorhabditis elegans , collated from the SGD database and from the literature [28] , [31] , [32] , [33] , [41] ( Supplementary Data 4 , Permutation test, empirical P -value<0.02). Finally, a recently published study has examined the correlation between gene expression measured in mice livers and lifespan extension across different diet regimens [42] . To further validate MTA’s performance in the context of mammals ageing, we applied it to two additional data sets describing gene expression levels of old and young liver mice [26] , [43] . We found that genes that are negatively correlated with lifespan (and thus, whose knockout will actually contribute to lifespan extension) indeed have significantly higher TSs than those genes that are positively correlated with lifespan (Wilcoxon’s test, P -value=0.003 for Sutton et al . [43] , and P -value=0.01 for Pearson et al . [26] ), further testifying for MTA’s significant predictive power. 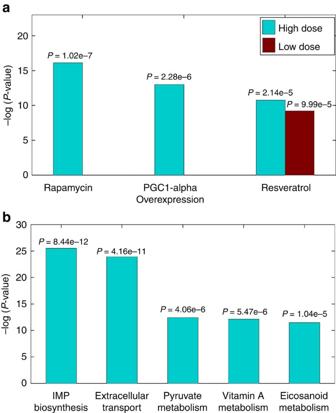Figure 5: Human ageing validation analysis. (a) Hypergeometric enrichment of the common knockout predictions set within genes whose expression is significantly reduced (t-test,P<0.05) following CR mimetic treatments. (b) Pathway enrichment analysis over the set of common knockout predictions, computed via hypergeometric test and corrected for multiple hypotheses using false discovery rate (α=0.05). Figure 5: Human ageing validation analysis. ( a ) Hypergeometric enrichment of the common knockout predictions set within genes whose expression is significantly reduced ( t -test, P <0.05) following CR mimetic treatments. ( b ) Pathway enrichment analysis over the set of common knockout predictions, computed via hypergeometric test and corrected for multiple hypotheses using false discovery rate ( α =0.05). Full size image Several pathways are enriched within the set of common knockout predictions ( Fig. 5b ), including the metabolism of eicosanoids. This pathway is known to be controlled by dietary fat and insulin and has widespread effects on many alterations occurring in ageing [44] . Further, resveratrol is thought to exert anti-inflammatory effects through the inhibition of two key eicosanoids enzymes, COX-1 and 5-lipoxygenase [44] (see Supplementary Note 1 , Supplementary Methods and Supplementary Fig. S4 for a detailed stoichiometric explanation underlying the eicosanoids metabolism prediction). MTA’s predictions also include the inosine monophosphate biosynthesis pathway whose inhibition was previously found to extend the CLS of yeast via the allosteric regulation of phosphofructokinase [31] (see Supplementary Note 1 and Supplementary Methods ). Predicting the effects of environmental perturbations To further validate MTA’s ability in predicting environmental perturbations, we applied it to predict the effects of nutrients’ dietary elimination on transforming the metabolic state of ageing muscle tissue (Methods). As described above, environmental perturbation is simulated by shutting down the nutrient’s transport reaction. Investigating the effects of combined knockouts in a transport reaction and in one of the top single (non-transport) knockouts reported in the previous section, we searched for synergistic combinations whose knockout TS is higher than the sum of scores obtained for each reaction alone. Highly ranked transport perturbations included the transport of methionine and tryptophan, whose deficiency in diet was shown to extend lifespan [45] , and of sucrose, whose dietary elimination was found to significantly affect the health and lifespan of elderly people [46] ( Supplementary Data 5 ). To examine the hypothesis that it is not the reduction of calories that mediates the extension of lifespan but the restriction of particular nutrient groups in the diet [47] , we clustered the transport reactions to the three major nutrient groups (amino acids, fatty acids and carbohydrates). In accordance with ref. 47 , we find that the dietary elimination of amino acids is predicted by MTA to be the most beneficial and that of carbohydrates is the least so (Hypergeometric test, P -value<0.004, Supplementary Fig. S5 ). Going beyond extant GSMM perturbation prediction methods that aim to identify a perturbation that could kill a target cell, we present a new approach for identifying drug targets that revert the metabolism of a diseased cell towards a healthier state. The predictive value of MTA is comprehensively demonstrated here via multiple existing perturbation data sets and by the identification of two predicted lifespan-extending genes in yeast. Notably, these genes could not be predicted by neither gene expression analysis alone nor by the commonly used prediction methods. Providing mechanistic explanations to their workings, we further show that in accordance with the model’s predictions, the knockout of the two lifespan-extending genes results in a significant elevation in ROS levels, potentially suggesting a hormetic mechanism, as previously shown by Masquita et al . [48] for H 2 O 2 . Of note, knockout of ADH2 was previously found to extend yeast CLS by driving metabolism away from acetic-acid production [49] , similar to the mechanism suggested by our flux analysis ( Fig. 3c ). A key prediction arising in the mammalian muscle tissue analysis involves the eicosanoids pathway, a suggested target of resveratrol. Indeed, a recent study by Timmers et al . [50] found that a 30-day supplementation of resveratrol results in a decrease in pathways linked to inflammation and an increase in the expression of mitochondrial oxidative phosphorylation. A stoichiometric analysis of aged human model (see Supplementary Fig. S4 ) complements these observations by providing a network level view of how the inhibition of the eicosanoids pathway works directly at the metabolic level to counteract ageing-related alterations. Further, a recently published paper by Park et al . [51] has reported that resveratrol inhibits the metabolic gene PDE4 . Interestingly, in three muscle data sets where the eicosanoids pathways came up as a predicted target by MTA [36] , [37] , [52] , the knockout of PDE4 is also highly ranked as a lifespan-extending target (within the top 3, 4 and 13%). Nevertheless, some limitations of MTA should be pointed out. First, although several CBM-based methods for inferring flux rates using gene expression data have been developed [9] , [10] , [14] , the correlation between these measurements is known to be limited [53] . Hence, gene expression levels serve only as cues for the likelihood that an enzyme supports the metabolic flux of its associated reaction. Nonetheless, as GSMMs encompass stoichiometric and thermodynamic information as well, these types of methods have shown to have a significant added value versus the raw gene expression in predicting metabolically related phenotypes. Second, metabolic models consist of metabolic enzymes alone (that is, regulatory and signalling molecules are outside the models’ scope), and its predictions are hence limited to the metabolic realm alone. Once more comprehensive models would be developed, this analysis could be easily extended to include non-metabolic genes as well. In addition, the human model is not specific to any tissue- or cell-type and hence lacks a predefined objective function. However, as previously shown [14] , the integration of gene expression data taken from a specific type of tissue allows one to overcome this hurdle and infer the most likely distribution of fluxes in a given tissue and state. Moreover, CBM analysis relies on the steady-state assumption and hence metabolite concentrations and enzyme activity levels cannot be calculated. Importantly, to calculate these measurements, detailed kinetic data are needed, information that is currently lacking on a genome-scale level. Finally, the fundamental challenge of identifying drug side effects is only partially addressed in this study by measuring the effect the predicted knockout may have on the production of key energy metabolites. Once a specific target has been successfully validated experimentally, its toxicity, selectivity and off-targets should be further examined. MTA is a generic approach that holds promise for many future applications. First, when a GSMM of the worm C. elegans will appear, the MTA analysis could be applied to study metabolic aspects of ageing in this model organism as well, complementing the accounts provided here for yeast and human models. In addition, MTA can be readily extended and applied to other types of perturbations, including partial or double knockouts. These types of analyses were left out of the scope of this paper because of the lack of sufficient validation that can support our findings. With the growing availability of gene expression data sets in a wide spectrum of metabolic-related disorders and the upcoming release of new and more refined models of human metabolism, MTA offers a systematic approach for identifying novel metabolic targets on a genome-scale. As such, we believe that the application of MTA can point to novel drug targets in a host of disorders where metabolism has an important role, including obesity, diabetes, neurodegenerative mitochondrial disorders and cancer. Importantly, the predicted drug targets may have lesser side effects than current drugs, as they do not only aim to remedy a disease-related disruption on a local level but rather aim to globally retrieve the network state back to a healthy one. A CBM of metabolism A metabolic network consisting of m metabolites and n reactions can be represented by a stoichiometric matrix S , where the entry S ij represents the stoichiometric coefficient of metabolite i in reaction j (ref. 54 ). A CBM imposes mass balance, directionality and flux capacity constraints on the space of possible fluxes in the metabolic network’s reactions through a set of linear equations Where v stands for the flux vector for all of the reactions in the model (that is, the flux distribution). The exchange of metabolites with the environment is represented as a set of exchange (transport) reactions, enabling a predefined set of metabolites to be either taken up or secreted from the growth media. The steady-state assumption represented in equation (1) constrains the production rate of each metabolite to be equal to its consumption rate. Enzymatic directionality and flux capacity constraints define lower and upper bounds on the fluxes and are embedded in equation (2). In the following, flux vectors satisfying these conditions will be referred to as feasible steady-state flux distributions. Gene knockouts are simulated by constraining the flux through the corresponding metabolic reaction to zero. Similarly, environmental perturbations are simulated by constraining the flux through the associated exchange reaction to zero. For each of the data set analysed here, we simulated the same media that was used in the experiment (that is, glucose minimal media for E. coli , YPD medium and synthetic complete for yeast, and RPMI and DMEM media for mouse and human cell lines). In the human muscle ageing data sets in which the media is unknown, a rich media in which all the uptakes are available was simulated. In addition, for modelling E. coli ’s metabolism we have used the iAF1260 model [55] , for yeast we have used the iMM904 model [56] and for modelling mouse human metabolism we have used Recon1 (ref. 12 ). The MTA Steps 1 and 2: Given a metabolic CBM model and gene expression levels of the source and target metabolic states, the following preprocessing steps are performed: (1) determining the baseline flux distribution at the source state ( v ref ). A flux distribution describing the source metabolic state based on its gene expression levels is obtained using iMAT (ref. 14 ). In brief, iMAT accepts as input a set of highly and lowly expressed genes based on gene expression levels. Next, it looks for a consistent enzyme activity solution where a maximal number of reactions that are considered highly expressed are indeed active and a maximal number of reactions that are considered lowly expressed are inactive. As our modelling technique takes into account other constrains such as thermodynamic and steady-state constrains, the solutions obtained by iMAT aims to capture modifications that go beyond the explicit gene expression information to capture post-transcriptional regulation effects. iMAT’s solution may not be unique as a space of alternative optimal solutions (in terms of its objective function) may exist. Therefore, we sample 2,000 different flux distributions that are all consistent with the reactions’ state of activity or inactivity defined in one of iMAT’s optimal solutions. The mean flux distribution obtained over the 2,000 samples then serves as an approximation of the source metabolic state and is denoted by v ref . (2) Analysing the source and target gene expression data to determine changed and unchanged genes and reactions. Applying the Student’s t -test to the source and target gene expression measurements given as input, we define genes that can be categorized into three sets: (a) genes whose expression did not change significantly; (b) genes whose expression is reduced in the source state compared with the target state (and therefore their flux activity should be elevated to transform the source back to the target metabolic state); and (c) genes whose expression is elevated in the source state compared with the target state (and therefore their flux activity should be reduced accordingly). Next, a detailed Boolean gene-to-reaction mapping (already embedded in the metabolic network model) is employed to map the above three sets of genes to determine the ‘changed’ state of their corresponding reactions in the model. Specifically, a reaction is considered to be elevated/reduced in two cases: (a) if it is catalysed by a complex of enzymes (an ‘and’ logical relation) and all of the genes encoding them were categorized as elevated or reduced, respectively, in the previous step; and (b) if it is catalysed by isoenzymes (an ‘or’ logical relation) and at least one of them was categorized as elevated or reduced, respectively. If a subset is categorized as elevated and another subset as reduced, the reaction is considered unchanged. In addition, in any other cases not specifically described here, the reaction is considered unchanged. Finally, a subset of the reactions in the metabolic network is considered reversible and can therefore carry both a positive and a negative flux rate. We, therefore, further categorize such reversible reactions that should be elevated or reduced to those whose flux should change in the forward or backward direction. Namely, reactions that should change in the forward direction are those that carry a positive flux in their reference state (according to v ref obtained in the first step) and were categorized as ‘elevated’ in the previous step, and those that carry a negative flux according to their reference state and were categorized as ‘reduced’ in the previous step. Reactions whose flux should change in the backward direction are determined in a complementary manner. Altogether, we obtain three different sets of reactions, those that did not change significantly (denoted as R S ) and those that did change significantly and should thus change in the forward or backward direction (denoted as R F and R B , respectively). Steps 3 and 4: As the desired TS (described below in step 4) is nonlinear, it could not have been used directly as the objective function. Hence, we chose to take a two-step heuristic approach: in step 3, we first minimize an objective function, which serves as conceptual proxy to what we are after (maximize the changes in the ‘changed’ reactions while keeping the flux on the ‘unchanged’ ones unchanged). Subsequently, in step 4, we rank the solutions obtained in step 3 by the (nonlinear) TS that, in practice, produces a more fined and accurate ranking of the perturbations’ predictions than the original objective. Below, we first describe the MIQP procedure taken in step 3, followed by a description of the TS applied in step 4. The MIQP formulation For each employed genetic or environmental perturbation v j , we formulated the following MIQP problem to find a steady-state flux distribution satisfying stoichiometric and thermodynamic constraints that (1) aims to keep the flux through reaction in R S as similar as possible to their value embedded in v r ef and (2) maximizes the number of reactions in R F and R B whose flux is elevated or reduced significantly in the desired direction, with respect to the flux in v ref : s.t The mass balance and thermodynamic (directionality) constraints are enforced in equations (1) and (2), respectively. The employed perturbation is enforced through equation (4). For each significantly changed reaction, the Boolean variables , y i represent whether the flux through the corresponding reaction is changed significantly (in either direction) or not. Specifically, a reaction that is required to change in the forward direction to transform from the source to the target metabolic state satisfies this demand if its flux is elevated by more than an ε with respect to the flux embedded in v ref (equations (5) and (6)). Similarly, a reaction that is required to change in the backward direction to perform a transformation between the two states satisfies this demand if its flux is reduced by more than an ε with respect to the flux in v ref (equations (7) and (8)). The ε value represents a significant flux change and can either be uniform across all changed reaction or reaction specific (see Methods and Supplementary Tables S1–S3 ). To comprehensively capture the transformation from one state to the other, the optimization function also aims at minimizing the change in flux rate with respect to v ref for reactions found in R S . Importantly, as flux rates may span several orders of magnitude and integer variables span only values of [0,1], the MIQP formulation contains an additional weighting parameter α in front of each term in the multiobjective function. The results presented in the main text are for the uniform choice ( α =0.66) but were found to be highly robust to α values in the range of 0.1–0.9 ( Supplementary Fig. S6 and Supplementary Tables S13–S21 ). Overall, the optimization problem minimizes the change in flux rate through the reactions that should remain unchanged while maximizing the number of reactions whose corresponding flux should differ significantly to transform from the source to the target state. The commercial CPLEX solver was used for solving MIQP problems on a Pentium-4 machine running Linux. The TS Relying on the optimization value obtained by MTA to rank the transformations induced by different perturbations is suboptimal, as the integer-based scoring of the changed reactions is coarse grained and does not distinguish between solutions achieving large flux alterations and those obtaining flux changes barely crossing the ε threshold. Therefore, we chose to quantify the success of a transformation by a scoring function based on the resulting flux distributions rather than on the optimization objective values themselves. First, we denote the resulting flux distribution obtained in a given MIQP solution (for a given reaction knockout) as v res . Second, reactions found in R F and R B are classified into two groups R success and R unsuccess , denoting whether they achieved a change in flux rate in the required direction (forward or backward) or not. The following scoring function is then used to assess the global change achieved by the employed perturbation: The numerator of this function is the sum over the absolute change in flux rate for all reactions in R success minus a similar sum for reactions in R unsuccess . The denominator is then the corresponding sum over reactions in R S (the reactions that should stay untransformed). Following perturbations achieving the highest scores under this definition are the ones most likely to perform a successful transformation by both maximizing the change in flux rate for significantly changed reactions and minimizing the corresponding change in flux of unchanged reactions. Using an alternative scoring function based on the Euclidean distance instead of absolute values yielded similar results. Although we believe that the TS score (equation (10)) is the right one to pursue from a biological point of view, optimizing it directly is a very difficult mathematical task. To accomplish that, one would need to develop a novel optimization algorithm for solving a mixed nonlinear programming problem, whose objective function is non-smooth and non-differentiable, requiring non-smooth optimization tools. Attempting such a solution directly would greatly complicate the problem, as one would need to add many variables and constraints. Further, the specific form of this ratio is actually dependent on the solution itself (as it evaluates R success and R unsuccess separately) making the entire task infeasible. In light of these evident difficulties, we have chosen to take a two-step approach in this study that is suboptimal yet tractable. Although the wild-type solution always achieves maximal values in terms of the original proxy objective function used in step 3 (by definition), it does not necessarily achieve high TSs (step 4). This is because the wild-type solution is the least constrained, and hence most of the solutions found in step 3 can be satisfied by achieving only a minimal epsilon change; those are obviously non-optimal from a biological standpoint as they do not really come close to the desired objective, and hence their TS score (in step 4) is suboptimal in many of the cases, correctly ruling them out as biologically viable solutions. Selection of thresholds in the MTA procedure As flux values vary significantly between different metabolic states, the specific choice of ε is determined in accordance with the data set in use, such that in each case only a statistically significant change is considered as a success. The MTA procedure involves the determination of two thresholds. The first is associated with the selection of the differentially expressed genes and is based on a t -test analysis. Here we consider statistically significant thresholds that are P -value<0.05. Within this group, the top 100–200 most differentially expressed reactions are defined as the set of ‘changed’ reactions. As demonstrated in the validation part of this study, this number of ‘changed’ reactions is sufficient for MTA to identify the correct perturbations; moreover, it allows us to obtain a tractable running time. Our results were found to be robust to different values within this range. The second threshold used is the ε parameter embedded in MTA’s formulation, denoting significant flux changes. As described above, The MTA procedure starts from estimating a baseline flux state distribution in the model using the iMAT analysis. This initial flux distribution is obtained using 2000 iMAT-based samples and its mean is denoted as v ref . To determine the ε value that best fits the initial distribution of fluxes and the specific set of reaction that should be changed, we implemented two different approaches: (a) using one threshold for all reactions: in this case, we apply a one-sided T -test for each changed reaction searching for an ε value that represents a significant change in flux rate with respect to the values in v ref . Specifically, ε is chosen such that for at least 70% of the reactions that should be changed (those found in R F and R B ), the values and , respectively, are significantly different ( P <0.05) from the values constituting (that is, the 2,000 values we sampled for each reaction in the network). The final ε chosen is the maximal one under which this percentage of reactions achieve a significant change; (b) use a specific threshold for each reaction: the same process as described in (a) is implemented with the difference of setting an ε representing a significant change ( P -value<0.05) for each reaction separately. Defining the set of simulated gene knockouts The metabolic models used in this study comprises a few thousands of reactions [12] , [55] , [56] . Notably, a subset of the reactions in each model (20–30%) is defined as dead end (that is, cannot carry metabolic flux because of the incompleteness of the model), and is therefore removed from the set of allowed knockouts. Similarly, essential reactions (knockout for which the growth was reduced by >80% of the maximal biomass) are excluded from the analysis in cases where biomass production is relevant. In addition, to further narrow down the number of simulated knockouts, we search for partially coupled reactions in the model [57] , whose deletion results with a similar outcome in terms of flux distribution. Finally, in the validation analyses, the set of simulated knockouts is composed of a member from each partially coupled set (including singleton sets). We refer to each reaction in a coupled set separately when performing enrichment analyses. Using MOMA for identifying transforming perturbations Similar to the procedure described above for obtaining the v ref description of the source metabolic state, to test MOMA’s predictions we produced an additional flux description vector, v res , based on the expression level of the target metabolic state. Then, MOMA’s objective function (that is, minimizing the Euclidean distance to a given wild-type flux distribution) following a perturbation is applied while using the v ref vector as the wild-type vector. Finally, the Euclidean distance between the obtained post-perturbation flux distribution and v res is evaluated. This distance ranks perturbations such that those that result with a smaller distance are considered the better transforming perturbations. Estimating the success rates of the yeast CLS experiment To estimate the success rate of the experimental procedure, we have used the information presented in Smith et al . [49] Specifically, this study describes the percentage of lifespan-extending genes found within a random group of genes as estimated via a screen-based experiment. The authors acknowledge that this type of experiment suffer from a high frequency of false positives and hence another (screen-based) experiment is next conducted to verify the results found in the first round. It is then that the authors report on a fraction of 3.5% lifespan-extending genes that can be found by random. Importantly, the experiments done in our study are small scale and do not have a high frequency of false positive. Therefore, we found that the 3.5% is the most appropriate number to assess the success of our results. As this fraction refers to the yeast genes in general, we additionally tried to estimate this fraction for metabolic lifespan-extending genes. Accordingly, we have analysed the SGD database and found that out of 104 CLS extending genes, 25 are metabolic ones that appear in the yeast metabolic model (24.04%). In addition, the fraction of metabolic genes (as found in the yeast metabolic model) out of the 6,000 yeast genes is 905/6,000 (15.08%). We therefore estimate that about 3.6% are metabolic lifespan-extending genes. A similar fraction to that has been reported by ref. 49 . Computing drug selectivity For each reaction found in the common knockout prediction set (see Supplementary Data 3 ), we examine the maximal production of ATP, NADP or NADPH (central energy metabolites). Our goal is to identify those predicted knockouts that reduce the production of these metabolites with respect to their wild-type production rates and mark them as non-selective drug targets. The analysis is performed in the following manner: (1) iMAT is applied using the ‘source’ gene expression data. (2) the maximal similarity between the expression and flux activity found by iMAT (that is, the number of satisfied integers) is added as an additional constraint to the optimization problem. (3) Then, under this constraint, the maximal production of the relevant metabolites is calculated in this wild-type baseline state. (4) Finally, for each predicted knockout, the maximal production of these energy metabolites is calculated again when the corresponding knockout reaction is additionally constrained to carry a zero flux. Notably, even when using lower similarity scores (for example, 80–90% of the maximal similarity score obtained by iMAT), our results remain essentially unchanged. Simulating environmental perturbations The metabolic model contains a set of reactions that allow the organism to take and secrete metabolites from and into the media. To simulate environmental perturbation and identify synergistic pairs, we focused on the top 10% predictions obtained by MTA in the four muscle tissue data sets analysed here. For each of these reactions, we examined the effect of its inhibition together with the inhibition of one media component. We then searched for those combinations that achieve a TS greater than the one achieved for the each of the reaction knockout alone. Focusing again on the top 10% of these pairs, we searched for those media metabolites that appear in at least two data sets. To investigate the hypothesis that it is not the reduction of calories that mediates the extension of lifespan, but the restriction of particular nutrient groups in the diet [47] , [58] , we clustered the transport reactions to the three major nutrient groups (amino acids, fatty acids and carbohydrates). We then produced a list indicating for each media metabolite, in how many of the four data sets it appeared in a synergistic pair. Finally, we calculated hypergeometric enrichment for each of the major nutrient groups within each of the groups found in the list described above (the groups are those media metabolites that appear in 4/3/2/1 data sets). Yeast strains All strains used in this study were BY4741 (MATa, his3Δ1, leu2Δ0, met15Δ0 and ura3Δ0). The deletion mutants were obtained from the yeast ORF knockout collection [59] . CLS assays CLS measurements were performed as described in refs 60 , 61 , with minor modifications. In short, strains were diluted from overnight cultures to OD 600 =0.1 in 10 ml fresh synthetic complete medium and incubated at 30 °C with 270 r.p.m. shaking till cultures reached stationary phase. After reaching stationary phase, aliquots from each culture were plated on YPD medium plates (1% yeast extract, 2% bacto peptone, 2% D -glucose and 2% agar) and colony forming unit was counted every 3 days. Each of the platings was done in triplicate and three distinct colonies of each strain were tested. ROS detection ROS detection was performed at several time points during the course of CLS. The days indication refers to the number of day passed since reaching stationary phase. O 2 − detection was carried out using dihydroethidium [62] , [63] . One micolitre of cell culture was centrifuged and resuspended in 1 ml PBS buffer plus 0.1% glycerol (4 °C). Dihydroethidium was added to final concentration of 5 μM and incubated at 30 °C for 30 min with shaking. Cells were centrifuged again and washed once with ice-cold PBS. For intracellular H 2 O 2 measurement 2′,7′-dichlorofluorescein diacetate [64] , [65] was used. One microlitre of cell culture was moved to eppendorf tube, H 2 O 2 was added to final concentration of 1 mM and tubes were incubated at 30 °C for 15 min with shaking. Cells were centrifuged, washed once and resuspended in ice-cold PBS. 2′,7′-dichlorofluorescein diacetate was added to final concentration of 10 μM and incubated at 28 °C for 1 h with shaking. Cells were centrifuged again and washed with ice-cold PBS. Probes florescence was measured by flow cytometry using Beckman Coulter Gallios Flow Cytometer. How to cite this article: Yizhak, K. et al . Model-based identification of drug targets that revert disrupted metabolism and its application to aging. Nat. Commun. 4:2632 doi: 10.1038/ncomms3632 (2013).